Conformational rearrangement of gastric H+,K+-ATPase induced by an acid suppressant Acid-related gastric diseases are associated with disorder of digestive tract acidification. The gastric proton pump, H + ,K + -ATPase, exports H + in exchange for luminal K + to generate a highly acidic environment in the stomach, and is a main target for acid suppressants. Here, we report the three-dimensional structure of gastric H + ,K + -ATPase with bound SCH28080, a representative K + -competitive acid blocker, at 7 Å resolution based on electron crystallography of two-dimensional crystals. The density of the bound SCH28080 is found near transmembrane (TM) helices 4, 5 and 6, in the luminal cavity. The SCH28080-binding site is formed by the rearrangement of TM helices, which is in turn transmitted to the cytoplasmic domains, resulting in a luminal-open conformation. These results represent the first structural evidence for a binding site of an acid suppressant on H + ,K + -ATPase, and the conformational change induced by this class of drugs. Current therapies to treat gastric acid-related diseases such as peptic ulcer or gastroesophageal reflux disease either prevent the stimulation of parietal cells or inhibit the final step in acid production [1] . The former is accomplished by antagonizing histamine H 2 receptors, and the latter by targeting the gastric proton pump, H + ,K + -ATPase. Proton pump inhibitors (PPIs) such as omeprazole abolish enzyme activity by covalently binding to the C813 residue of gastric H + ,K + -ATPase to alleviate the painful symptoms [2] . A new class of acid suppressants is undergoing clinical trials to provide a more rapid and efficient cure than achieved by PPIs. Unlike PPIs, SCH28080 (ref. 3 ) and its derivatives inhibit H + ,K + -ATPase noncovalently in a K + -competitive manner from the luminal side of the enzyme, and are thus called potassium-competitive acid blockers (P-CABs) [4] . As inhibition by omeprazole and SCH28080 is mutually exclusive [5] , the binding region of these two compounds seems to overlap. H + ,K + -ATPase mediates the electro-neutral exchange of H + and K + across the parietal cell membrane accompanying ATP hydrolysis [6] . Characteristic of all P-type ATPases, vectorial cation transport is accomplished by cyclical conformational changes between the two principal reaction states (E 1 and E 2 ) and their corresponding phosphoenzyme intermediates (E 1 P and E 2 P), which are formed by reversible auto-phosphorylation of an aspartate residue in the invariant 385 DKTG motif [7] . According to the Post-Albers-type reaction scheme [8] , cytoplasmic-facing E 1 and luminal-facing E 2 states show high affinity for H + and K + , respectively. H + ,K + -ATPase consists of two subunits. The catalytic α-subunit is homologous to the other P2-type ATPases [9] such as Na + ,K + -ATPase and sarco(endo)plasmic reticulum Ca 2+ -ATPase (SERCA). It comprises ten transmembrane (TM) helices (M1–M10), in which cation-binding sites are located, and three cytoplasmic domains, the nucleotide-binding (N), phosphorylation (P) and actuator (A) domains [10] . In addition to the α-subunit, H + ,K + - and Na + ,K + -ATPase require an accessory β-subunit, which is important for K + -occlusion [11] , [12] and the functional expression of the complex [13] . The H + ,K + -ATPase β-subunit is also important for blocking reversion of the transport cycle by stabilizing the E 2 P conformation with its amino terminus [14] , [15] . Despite the close similarity between the primary structures of the H + ,K + - and Na + ,K + -ATPase α-subunits (63% identity), their various specific inhibitors (such as SCH28080 for H + ,K + -ATPase or ouabain for Na + ,K + -ATPase) strictly discriminate their binding site in each target molecule. Yet, their inhibitory nature is quite similar, because both inhibitors preferentially bind in a K + -competitive manner to the extracellular side of the E 2 P conformation [3] , [16] , [17] , [18] . Furthermore, some overlap between the binding sites is expected, because substitution of seven amino acids located in M4 and M5 renders H + ,K + -ATPase ouabain-sensitive [19] . The recent X-ray structure of Na + ,K + -ATPase with bound K + and ouabain shows the inhibitor-binding site in detail [20] . Although the structure represents ouabain binding in the low-affinity mode due to antagonism between ouabain and K + , the authors predicted the conformational change required for the high-affinity ouabain binding based on the luminal-open conformation of the beryllium fluoride (BeF)-bound SERCA E 2 BeF structure [21] . Despite a number of biochemical [2] , [22] and mutagenesis studies [23] , [24] , [25] , [26] , [27] , [28] , [29] as well as computational approaches [27] , [28] , [29] for the interaction between the H + ,K + -ATPase and its inhibitors, however, the detailed structural information has not been elucidated. Here, we show for the first time structural evidence for the SCH28080-binding site of H + ,K + -ATPase and the conformational rearrangement induced by the binding of SCH28080, which is a P-CAB prototype currently under development. The binding of SCH28080 to the E 2 P conformation cannot be explained by a simple 'lock and key' model, because the binding induces the widely opened luminal cavity formed in the TM domain, which itself requires the conformational change of the whole enzyme including the cytoplasmic domains and connecting linkers. Conversely, as shown by crystal structures of SERCA in various reaction states [21] , [30] , the phosphorylation/dephosphorylation-driven rearrangement of the cytoplasmic domains induces open–close movements of the TM helices. Therefore, the overall conformational change required for formation of the luminal-open structure is conserved, at least among H + ,K + -ATPase and SERCA, and most likely such tightly coupled motion between two highly separated parts of the enzyme (that is, cytoplasmic domains and TM helices) provides a framework for all of P-type ATPases. Three-dimensional structure of SCH28080-bound H + ,K + -ATPase To elucidate the inhibitor-binding site and induced conformational changes of H + ,K + -ATPase, we prepared two-dimensional (2D) crystals in the presence of the phosphate analogue BeF and SCH28080, a P-CAB prototype. Similar to the previously reported BeF-bound 2D crystals [31] , large tubular crystals were formed in the presence of SCH28080 ( Supplementary Fig. S1a ), and were analysed by electron crystallography using cryo-electron microscopy [32] ( Supplementary Fig. S1 and Supplementary Table S1 ). The final three-dimensional electron microscopic density map (EM density map) was calculated to 7 Å resolution ( Fig. 1a , Supplementary Movie S1 ). Consistent with the crystallization conditions, the overall structure of the present EM density map ( Fig. 1a ) shows characteristic features of the ADP-insensitive E 2 P conformation to which SCH28080 is preferentially bound ( Supplementary Fig. S2 ) [16] . The BeF-bound phosphorylation site (Asp385) at the P domain is covered by the A domain, and the ADP-bound N domain is separated from the P domain, thus the bound phosphate analogue seems to be isolated from both ADP and the bulk solution ( Supplementary Fig. S3 ). The structure is not identical, however, to that of previously reported pseudo-E 2 P states [14] , [31] (as both the aluminium fluoride (AlF)-bound E 2 AlF and the BeF-bound E 2 BeF structures of H + ,K + -ATPase are indistinguishable at the currently achieved resolution, they are abbreviated as E 2 P* unless otherwise stated). Therefore, the present structure is designated as an SCH28080-bound pseudo-E 2 P state, (SCH)E 2 BeF, which represents a conformation different from that of the inhibitor-free E 2 P* structures described later. Because of the similarity in their primary sequences, overall conformations, and representative reaction states (inhibitor-bound E 2 P state), we used the ouabain-bound Na + ,K + -ATPase [20] atomic model (PDB ID: 3A3Y ) as a starting template for the homology model. The EM density map allowed us to determine the position of the individual helices in the TM domain, as well as in the cytoplasmic domains, and we successfully generated a homology model of H + ,K + -ATPase by fitting them into the EM density map as rigid bodies. 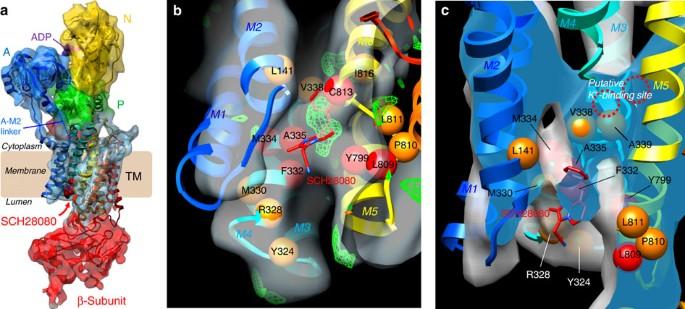Figure 1: SCH28080-bound E2P structure of H+,K+-ATPase analysed at 7 Å resolution. (a) Overall structure of the H+,K+-ATPase. The molecular surface represents the EM density map (contoured at 1σ) with a superimposed homology model of H+,K+-ATPase (ribbon). Bound SCH28080 at the luminal cavity and ADP at the N domain are shown as red and purple spheres, respectively. The yellow–brown box indicates the approximate location of the lipid bilayer. Colour code: A domain, blue; P domain, green; N domain, yellow; TM domain, light blue (surface); β-subunit, red. Colour of the TM helices of the homology model gradually changes from M1 (blue) to M10 (red). As described in the text, the homology model does not contain the A-M2 linker (dotted line in blue). (b) SCH28080-binding site viewed from the luminal side (red arrow ina). The amino acids important for SCH28080 affinity are indicated as spheres (red, more than 10 times lower affinity; orange: 3–10 times lower, based on mutagenesis studies)20,21,22,23,24,25,26,27,28to show their locations on the chain trace of the homology model (ribbon, colour codes as ina). Green mesh represents the excess density (that is, [EM density map (1σ, white surface)]−[homology model], see text for details), showing good fit with the predicted position of SCH28080 by the docking simulation (stick model, see alsoFig. 2aand Discussion). (c) A cross-section of the TM region perpendicular to the membrane plane. The EM density map contoured at 1σ is shown as a white surface, and the sectional surface is shown in blue. Dotted spheres indicate K+-binding sites of the Na+,K+-ATPase20to show the approximate location of the cation binding site on the H+,K+-ATPase, yet these ions are not resolved in the present (SCH)E2BeF structure because of the limited resolution of the EM density map and K+-free conditions for the 2D crystallization. The M6 helix was omitted for clarity. Bound SCH28080 (red stick, position predicted by the docking simulation) is found at the centre of the luminal cavity, apparently blocking the K+-entry pathway from the luminal side of the membrane. Figure 1: SCH28080-bound E 2 P structure of H + ,K + -ATPase analysed at 7 Å resolution. ( a ) Overall structure of the H + ,K + -ATPase. The molecular surface represents the EM density map (contoured at 1σ) with a superimposed homology model of H + ,K + -ATPase (ribbon). Bound SCH28080 at the luminal cavity and ADP at the N domain are shown as red and purple spheres, respectively. The yellow–brown box indicates the approximate location of the lipid bilayer. Colour code: A domain, blue; P domain, green; N domain, yellow; TM domain, light blue (surface); β-subunit, red. Colour of the TM helices of the homology model gradually changes from M1 (blue) to M10 (red). As described in the text, the homology model does not contain the A-M2 linker (dotted line in blue). ( b ) SCH28080-binding site viewed from the luminal side (red arrow in a ). The amino acids important for SCH28080 affinity are indicated as spheres (red, more than 10 times lower affinity; orange: 3–10 times lower, based on mutagenesis studies) [20] , [21] , [22] , [23] , [24] , [25] , [26] , [27] , [28] to show their locations on the chain trace of the homology model (ribbon, colour codes as in a ). Green mesh represents the excess density (that is, [EM density map (1σ, white surface)]−[homology model], see text for details), showing good fit with the predicted position of SCH28080 by the docking simulation (stick model, see also Fig. 2a and Discussion). ( c ) A cross-section of the TM region perpendicular to the membrane plane. The EM density map contoured at 1σ is shown as a white surface, and the sectional surface is shown in blue. Dotted spheres indicate K + -binding sites of the Na + ,K + -ATPase [20] to show the approximate location of the cation binding site on the H + ,K + -ATPase, yet these ions are not resolved in the present (SCH)E 2 BeF structure because of the limited resolution of the EM density map and K + -free conditions for the 2D crystallization. The M6 helix was omitted for clarity. Bound SCH28080 (red stick, position predicted by the docking simulation) is found at the centre of the luminal cavity, apparently blocking the K + -entry pathway from the luminal side of the membrane. Full size image SCH28080-binding site As predicted by earlier homology modelling of H + ,K + -ATPase [25] , [26] , [27] , [28] , [29] together with mutagenesis studies, the density responsible for bound SCH28080 was found in the luminal cavity ( Fig. 1b ). The subtraction map (that is, [EM density map]−[homology model], green mesh in Fig. 1b , Fig. 2a,b ) clearly shows an excess density in the centre of the luminal cavity. The density is located near the luminal part of M4, M5 and M6 in the luminal ion entry path ∼ 12 Å from the ion-binding site ( Fig. 1c ), consistent with the K + -competitive inhibition mode of SCH28080 (refs 3 , 17 ). The density is also predicted to be surrounded by several important amino acids [26] , [27] , [28] for SCH28080 affinity, including F332, A335, Y799, L809 and C813 ( Fig. 1b,c ). Molecular docking simulation of SCH28080 to the H + ,K + -ATPase homology model suggested that its potential binding site is close to the observed density ( Fig. 2a ), consistent with many of the earlier studies described above. 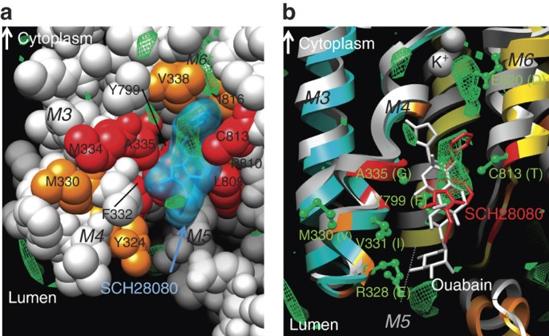Figure 2: SCH28080-binding site. (a) Predicted binding mode of SCH28080 (blue stick with transparent surface rendering) to the homology model (spheres) determined by docking simulations. The green mesh shows the subtracted density and amino acids important for the SCH28080-binding are highlighted in red or orange (as shown inFig. 1b). The calculated binding site of SCH28080 fits well into the homology model as well as the experimentally determined density (green mesh), supporting the reliability of the proposed (b) Comparison between SCH28080- (red stick) and ouabain (white stick)-binding sites. The ribbon models represent the homology model of H+,K+-ATPase (SCH)E2BeF (colour as inFig. 1a, positions for several important amino acids are marked in red or orange as inFig. 1b) and the X-ray structure of ouabain-bound Na+,K+-ATPase (grey)20. Indicated in green (ball and stick representation) are side chains, which must be mutated for the formation of an ouabain-sensitive H+,K+-ATPase19. White spheres represent bound K+ions in the Na+,K+-ATPase structure. The overlap between these two specific inhibitors seems to be consistent with their similar modes of inhibition. In both figure panels, helices M1 and M2 were omitted for clarity. Figure 2: SCH28080-binding site. ( a ) Predicted binding mode of SCH28080 (blue stick with transparent surface rendering) to the homology model (spheres) determined by docking simulations. The green mesh shows the subtracted density and amino acids important for the SCH28080-binding are highlighted in red or orange (as shown in Fig. 1b ). The calculated binding site of SCH28080 fits well into the homology model as well as the experimentally determined density (green mesh), supporting the reliability of the proposed ( b ) Comparison between SCH28080- (red stick) and ouabain (white stick)-binding sites. The ribbon models represent the homology model of H + ,K + -ATPase (SCH)E 2 BeF (colour as in Fig. 1a , positions for several important amino acids are marked in red or orange as in Fig. 1b ) and the X-ray structure of ouabain-bound Na + ,K + -ATPase (grey) [20] . Indicated in green (ball and stick representation) are side chains, which must be mutated for the formation of an ouabain-sensitive H + ,K + -ATPase [19] . White spheres represent bound K + ions in the Na + ,K + -ATPase structure. The overlap between these two specific inhibitors seems to be consistent with their similar modes of inhibition. In both figure panels, helices M1 and M2 were omitted for clarity. Full size image Another density can be found near the putative K + -binding site ( Fig. 2b , upper density). The density is too far, however, to be contributed to amino acids important for SCH28080 binding [2] , [28] , such as A335 (12.3 Å, the distance between C α carbon of this residue and the centre of the density) or C813 (9.1 Å) compared with their close proximity to the proposed binding site (5.4 Å for both A335 and C813). Furthermore, many reported mutations can affect inhibitor affinity without affecting K + affinity [25] , [26] , [28] , [29] , showing that the competitive nature of the SCH28080 is due to mutual exclusion and not to direct overlap of the inhibitor and ion binding sites. Therefore, we conclude that the upper density in Figure 2b is unlikely to represent a bound SCH28080 molecule. It is notable that the lower density in Figure 2b does not cover the complete SCH28080 molecule. Because SCH28080 is a non-chiral molecule, disorder or rotation of one part of the molecule relative to the other might be responsible for insufficient determination of its density. Rearrangement of TM helices induced by SCH28080 binding Comparison between the E 2 P* and (SCH)E 2 BeF structures of H + ,K + -ATPase reveals that binding of SCH28080 induces the rearrangement of, mostly, the M1–M4 helices at the luminal side of the enzyme ( Fig. 3 ). Although all TM helices are located in similar positions on the cytoplasmic side of the membrane ( Supplementary Fig. S4a,b ), M3 and M4 bend outwardly at the luminal membrane interface ( Fig. 3a , Supplementary Fig. S4c ). This difference, which is also observed in the ouabain-bound Na + ,K + -ATPase structure [20] , clears space at the luminal cavity to create the binding site for SCH28080, where M4 locates in the H + ,K + -ATPase E 2 P* structure ( Fig. 3a ). At the same time, the helix bundle of M1 and M2 moves towards the cytoplasmic side along with an outwards movement of M4 ( Fig. 3 ). As a consequence, M1 and M2 come closer and apparently restrict the SCH28080-binding site ( Fig. 3a ), which is consistent with the slow dissociation of SCH28080 (ref. 16 ), the fourfold lower affinity of L141C mutant located in M2 (ref. 28 ) ( Fig. 1b,c ), and the photoaffinity labelling between the M1–M2 segment and a SCH28080 derivative [22] . Such an inwards swinging motion of the M1–M2 bundle ( Fig. 3a,b ) has not been observed in the Na + ,K + -ATPase structure with bound ouabain in the low-affinity mode ( Supplementary Fig. S5 ), but has been predicted in the high-affinity ouabain-binding model based on the SERCA E 2 BeF structure [20] , [21] , which is consistent with the previously reported important contribution of the M1–M2 segment to the high-affinity ouabain binding [33] . Therefore, the M1–M2 movement observed in the H + ,K + -ATPase structure ( Supplementary Fig. S5 ) seems to be commonly involved in the formation of the high-affinity inhibitor-binding pocket on both closely related ATPases. Overall, this rearrangement of the TM helices of the H + ,K + -ATPase results in the luminal-open conformation, similar to that observed in the SERCA E 2 BeF structure [21] , [30] , which presumably allows for the release of bound Ca 2+ . 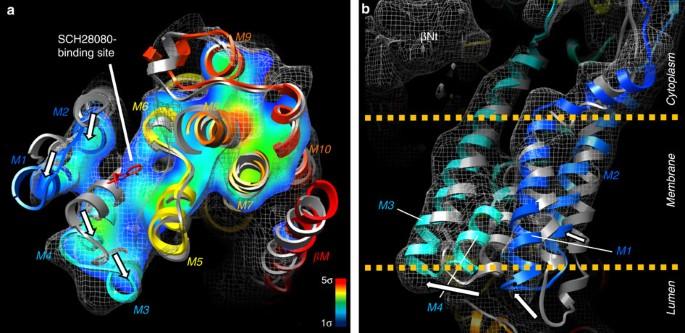Figure 3: Rearrangement of TM helices induced by SCH28080 binding. (a) Comparison of the TM helices between E2AlF and (SCH)E2BeF structures. A cross-section of the luminal TM region parallel to the membrane plane is viewed from the luminal side of the membrane. Mesh represents the EM density map (1σ) of (SCH)E2BeF, with homology models of (SCH)E2BeF (colour ribbons as inFig. 1a) and E2AlF (grey ribbon)14superimposed. A cross-section parallel to the membrane plane displays the contour level at the indicated plane (colour gradually changes from blue (1σ) to red (5σ) as indicated in the figure). White arrows indicate the conformational change of M1–M4 induced by the SCH28080 binding (red stick as inFig. 1b). The position of the slice is indicated as a red box inSupplementary Fig. S4. (b) A view of the M1–M4 region perpendicular to the membrane plane showing inwardly swinging movement of the M1–M2 helix bundle (blue ribbon) along with an outwards movement of M3–M4 (cyan ribbon) compared with the E2AlF homology model (grey ribbon). Dotted lines indicate the approximate position of the lipid bilayer. Figure 3: Rearrangement of TM helices induced by SCH28080 binding. ( a ) Comparison of the TM helices between E 2 AlF and (SCH)E 2 BeF structures. A cross-section of the luminal TM region parallel to the membrane plane is viewed from the luminal side of the membrane. Mesh represents the EM density map (1σ) of (SCH)E 2 BeF, with homology models of (SCH)E 2 BeF (colour ribbons as in Fig. 1a ) and E 2 AlF (grey ribbon) [14] superimposed. A cross-section parallel to the membrane plane displays the contour level at the indicated plane (colour gradually changes from blue (1σ) to red (5σ) as indicated in the figure). White arrows indicate the conformational change of M1–M4 induced by the SCH28080 binding (red stick as in Fig. 1b ). The position of the slice is indicated as a red box in Supplementary Fig. S4 . ( b ) A view of the M1–M4 region perpendicular to the membrane plane showing inwardly swinging movement of the M1–M2 helix bundle (blue ribbon) along with an outwards movement of M3–M4 (cyan ribbon) compared with the E 2 AlF homology model (grey ribbon). Dotted lines indicate the approximate position of the lipid bilayer. Full size image Conformational change of the whole-enzyme strcuture The conformational change observed in the TM region is transmitted to the cytoplasmic part of the enzyme, mostly by connecting linker between the A domain and M2 (A-M2 linker, Fig. 4a–c ). Because of the observed movement of the M1–M2 bundle on SCH28080 binding ( Fig. 3b ), the A-M2 linker forms an upright rod-like conformation separate from the P domain in the (SCH)E 2 BeF structure ( Fig. 4b,c ), which is in distinct contrast to its configuration in E 2 P* ( Fig. 4a ) [14] , [31] . It should be noted that the A-M2 linker is missing in this (SCH)E 2 BeF homology model ( Fig. 4b,c , dashed line, F161–P175), because of the large difference between the EM density map and the starting template structure (ouabain-bound Na + ,K + -ATPase [20] ). Comparison of the A-M2 linker conformations among several known structures of other P2-type ATPases [20] , [21] , [30] , however, reveals that it can assume mainly two conformations ( Supplementary Fig. S6 ). The A-M2 linker is unwound in structures of the E 2 AlF conformation of the H + ,K + -ATPase and SERCA, and the E 2 MgF structure of Na + ,K + -ATPase with bound ouabain, but a continuous α-helical conformation in SERCA E 2 BeF [21] , and the latter fits well into the EM density map of H + ,K + -ATPase (SCH)E 2 BeF ( Supplementary Fig. S6 ). Thus, it is highly likely that this part of M2 continues as an α-helix beyond the cytoplasmic interface of the membrane. As the mutation of Q159 found at the cytoplasmic end of M2 has a fourfold lower affinity [29] for SCH28080 despite its location on the opposite side of the membrane 35 Å away from the SCH28080-binding site ( Fig. 4b,c ), the conformational change of the A-M2 linker is important for the formation of the SCH28080-binding site. As suggested by SERCA structures [21] , the α-helix formation of the A-M2 linker may shorten the distance between the A domain and M2, inducing the observed location of the M1–M2 helix bundle ( Fig. 3 ). Therefore, also for the H + ,K + -ATPase, the A-M2 linker works as a determinant for the position of the M1–M2 bundle ( Supplementary Fig. S6 ), which is likely to be coupled with the outwards movement of the M3–M4 helices. 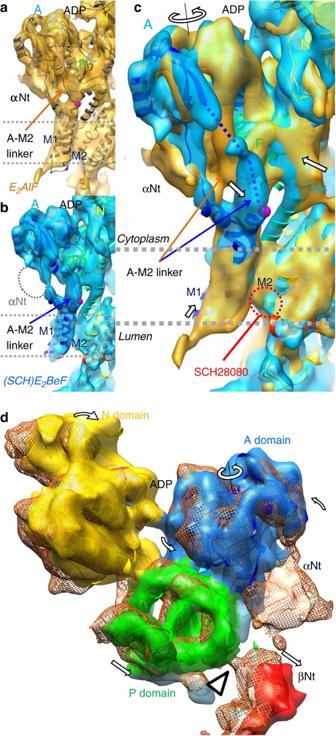Figure 4: SCH28080-induced conformational changes at the cytoplasmic part of the H+,K+-ATPase. (a–c) Close-up view of the A-M2 linker in E2AlF (a), (SCH)E2BeF (b) and their comparison (c). Each surface (white for E2AlF, blue for (SCH)E2BeF) and ribbon model (grey for E2AlF, colour for (SCH)E2BeF is as inFig. 1a) represents the EM density map and homology model of the corresponding structures, respectively. The magenta sphere indicates Q159, which on mutation to Asn showed fourfold lower affinity for SCH28080. The A-M2 linker of E2AlF or (SCH)E2BeF is indicated by orange or blue arrows, respectively, yet the (SCH)E2BeF homology model does not contain this part (dotted blue line inb,c, see also text). Note that density for the N-terminal domain of the α-subunit (αNt) is absent in the (SCH)E2BeF structure (b, dotted circle) in contrast to the E2AlF structure (a). (d) Conformational change of the cytoplasmic domains. The surface shows the EM density map of (SCH)E2BeF with its homology model superimposed (colour codes as inFig. 1a: A domain, blue; P domain, green; N domain, yellow; TM domain, light blue). Orange mesh represents the E2AlF EM density map. It should be noted that the inter-subunit interaction between the P domain and the N-terminal tail of the β-subunit (βNt) observed in the E2AlF structure is not present in the (SCH)E2BeF structure (arrowhead, see text for details). All the EM density maps are drawn with a 1σ contour level. White arrows in all panels indicate observed conformational changes during the E2AlF→(SCH)E2BeF transition. Figure 4: SCH28080-induced conformational changes at the cytoplasmic part of the H + ,K + -ATPase. ( a – c ) Close-up view of the A-M2 linker in E 2 AlF ( a ), (SCH)E 2 BeF ( b ) and their comparison ( c ). Each surface (white for E 2 AlF, blue for (SCH)E 2 BeF) and ribbon model (grey for E 2 AlF, colour for (SCH)E 2 BeF is as in Fig. 1a ) represents the EM density map and homology model of the corresponding structures, respectively. The magenta sphere indicates Q159, which on mutation to Asn showed fourfold lower affinity for SCH28080. The A-M2 linker of E 2 AlF or (SCH)E 2 BeF is indicated by orange or blue arrows, respectively, yet the (SCH)E 2 BeF homology model does not contain this part (dotted blue line in b , c , see also text). Note that density for the N-terminal domain of the α-subunit (αNt) is absent in the (SCH)E 2 BeF structure ( b , dotted circle) in contrast to the E 2 AlF structure ( a ). ( d ) Conformational change of the cytoplasmic domains. The surface shows the EM density map of (SCH)E 2 BeF with its homology model superimposed (colour codes as in Fig. 1a : A domain, blue; P domain, green; N domain, yellow; TM domain, light blue). Orange mesh represents the E 2 AlF EM density map. It should be noted that the inter-subunit interaction between the P domain and the N-terminal tail of the β-subunit (βNt) observed in the E 2 AlF structure is not present in the (SCH)E 2 BeF structure (arrowhead, see text for details). All the EM density maps are drawn with a 1σ contour level. White arrows in all panels indicate observed conformational changes during the E 2 AlF→(SCH)E 2 BeF transition. Full size image According to this SCH28080-induced conformational change in the A-M2 linker, the A domain is rotated ∼ 20° around an axis perpendicular to the membrane plane ( Fig. 4c,d , see also Supplementary Fig. S7 ), and the P domain is shifted along with the A domain ( Fig. 4d , see discussion ). These movements of cytoplasmic domains are also found in SERCA structures during the transition from the E 2 AlF to the E 2 BeF states [21] ( Supplementary Fig. S7 ). Consequently, the overall conformation of the H + ,K + -ATPase (SCH)E 2 BeF shows a conformation similar to SERCA E 2 BeF, including luminal-open TM helices, an α-helical structure of the A-M2 linker, and the arrangement of cytoplasmic domains. Therefore, the conformational rearrangement in the cytoplasmic region is tightly coupled with that in the TM domain, the latter of which is essential for the high-affinity binding of SCH28080 to the H + ,K + -ATPase (see also Discussion). In contrast to the previously reported E 2 AlF structure [14] , the cytoplasmically exposed N-terminal tail of the β-subunit (βNt) is detached from the P domain of the α-subunit in the (SCH)E 2 P BeF structure ( Fig. 4d ). The βNt in the E 2 AlF structure is in close proximity to the N-terminal part of the α-subunit (αNt), which is completely absent in the (SCH)E 2 BeF presumably because of its disorder ( Fig. 4d ). Because the αNt structure contributes crystal contacts with a neighbouring molecule in the E 2 AlF structure in contrast to the present (SCH)E 2 BeF structure, its disorder might be related to the inherent flexibility of the αNt. The spatial proximity between the N-termini of the α- and β-subunits, however, suggests that the αNt is involved in the regulation of the unique inter-subunit interaction between the βNt and the P domain. The predicted orientation of SCH28080 from the docking simulation highly overlaps with the experimental density ( Fig. 1b ), thus further supporting the reliability of the proposed binding site. In the predicted binding model ( Fig. 2a ), the SCH28080 molecule is tightly coordinated by several important amino acids, including F332 (ref. 28 ), A335 (ref. 28 ), Y799 (ref. 27 ), L809 (ref. 26 ), C813 (covalent-binding site of PPIs) [2] , [26] , and L141 (not shown in Fig. 2a ) [29] and V338 (ref. 28 ), I816 (ref. 26 ). The tight binding mode of SCH28080 seems to be consistent with its high-affinity binding. This SCH28080-binding site on H + ,K + -ATPase largely overlaps with the ouabain-binding site on Na + ,K + -ATPase [20] ( Fig. 2b ), in agreement with their similar mode of inhibition, and the position of seven amino acids, which must be mutated to generate a ouabain-sensitive H + ,K + -ATPase ( Fig. 2b ) [19] , supporting the reliability of the proposed SCH28080-binding site. It should be noted that we used the homology model with a truncated luminal loop between M1 and M2 (S129–D136) for the final molecular docking simulation. When we performed molecular docking using a 'full-length' homology model, the binding site shifted towards the M1–M2 loop compared with the 'final' model. That shifted binding site is inconsistent with our EM density map as well as earlier mutation studies, and was thus rejected as a binding site. As the M1–M2 loop is invisible in the present EM density map ( Fig. 1b ), this part may be disordered and presumably does not contribute to SCH28080 binding, as suggested by a previous study using chimeric enzymes between H + ,K + and Na + ,K + -ATPase [24] . Structural comparison between the SCH28080-bound H + ,K + -ATPase and the ouabain-bound Na + ,K + -ATPase [20] reveals important similarities and differences in the arrangement of their TM helices ( Supplementary Fig. S5 ). Highly overlapped position of each inhibitor bound to M4 interface suggests that the outwards movement of the M3–M4 bundle relative to their location in the E 2 P* conformation ( Fig. 3a ) is the primary event for the inhibitor binding on each closely related ATPase. There was, however, a significant difference in the orientation of the M1–M2 bundle (white arrows in Supplementary Fig. S5 ), in contrast to the similar arrangement of other TM helices. The observed orientation of M1–M2 bundle close to bound SCH28080 in H + ,K + -ATPase EM structure seems to accommodate the bound SCH28080 molecule, thus contributing to its high-affinity binding. This observation further supports the prediction for the high-affinity ouabain-binding mode of Na + ,K + -ATPase [20] . Although the bound SCH28080 is apparently accessible from the luminal bulk solution ( Fig. 1b ), it is likely to be tightly coordinated in its binding cavity ( Fig. 2 ). Therefore, such an open–close movement of the M1–M2 bundle ( Supplementary Fig. S5 ) as well as M3–M4 ( Fig. 3a ), during thermal fluctuation of the enzyme seems to be important for deep introduction of the inhibitor in its binding pocket, and for locking it in the appropriate position. As described in the results section, SCH28080 binding induces a luminal-open conformation of H + ,K + -ATPase. The overall conformation of H + ,K + -ATPase (SCH)E 2 BeF is thus similar to that of SERCA E 2 BeF (refs 20 , 21 ), in which the luminal ion gate is widely opened to release Ca 2+ . Therefore, the observed luminal-open feature of H + ,K + -ATPase (SCH)E 2 BeF is suggestive for the exchange of transporting H + /K + at the luminal side of the membrane, as the translocation of the cations, at least K + , requires physical paths to their binding site in H + ,K + -ATPase. As previously demonstrated, even using BeF alone, the H + ,K + -ATPase E 2 BeF structure shows the luminal-closed conformation [31] in contrast to the Ca 2+ -releasing luminal-open conformation of SERCA E 2 BeF. Accordingly, in the case of H + ,K + -ATPase, the luminal-closed conformation found in E 2 P* structure seems to be energetically more favourable than the present luminal-open conformation, which is constrained by SCH28080 binding. Therefore, we speculate that the luminal-open conformation without SCH28080 can be formed, but is short-lived, transiently appearing during thermal fluctuation when cations are exchanged at the luminal side of the membrane. Considering the K + -competitive nature of SCH28080 (refs 3 , 16 , 17 ) and its structural feature described above, it is likely that the present structure partially reflects a K + -binding event, which significantly accelerates the dephosphorylation of E 2 P to proceed with the transport cycle. In addition, the inter-subunit interaction between βNt and the P domain in the E 2 AlF structure has been proposed to function as a 'ratchet' to prevent a physiologically unfavourable reverse reaction (namely, E 1 P formation from E 2 P) by tethering the P domain in suitable position for the E 2 P formation [14] , thus stabilizing the E 2 P conformation [15] . Therefore, the disruption of the inter-subunit interaction between the βNt and the P domain observed here might occur when the reaction cycle proceeds in the forwards direction from E 2 P. Further structural and functional analyses of different reaction intermediates (that is, K + -bound E 2 P or K + -occluded E 2 ) are required, however, for a better understanding of the βNt function. Such conformational preference may be advantageous for the prevention of the H + reverse flow in the highly acidic environment of the stomach lumen. Two-dimensional crystallization and image analysis H + ,K + -ATPase-containing membrane fraction purified from pig stomach [34] , [35] (8 mg ml −1 of protein) was solubilized for 10 min on ice with 6.5 mg ml −1 octaethyleneglycol dodecylether (C 12 E 8 , Nikko Chemical) in 40 mM MES, 20 mM Mg(CH 3 COO) 2 , 5 mM ATP, 10% (v/v) glycerol and 3 mM dithiothreitol (DTT), at pH 5.5 adjusted by Tris buffer. The insoluble material was removed by ultracentrifugation at 186,000 g for 20 min, and the supernatant was mixed with dioleoylphosphatidylcholine (Avanti) at a lipid-to-protein ratio (w/w) ranging from 0.95 to 1.15. The samples were then placed in 10 μl microdialysis buttons (Hampton Research) using a dialysis membrane with a molecular weight cut-off of 25 kDa (SPECTRA/Pro #7, SPECTRUM), and first dialysed on ice for 36 h against 10 mM MES, 10% (v/v) glycerol, 10 mM MgCl 2 , 1 mM BeSO 4 , 4 mM NaF, 1 mM ADP, 3 mM DTT and 1 μM SCH28080 at pH 5.5 adjusted by Tris buffer, and then at 3 °C for 12–16 days against 20 mM propionate, 1 mM MgCl 2 , 1 mM BeSO 4 , 4 mM NaF, 1 mM ADP, 3 mM DTT and 0.1 mM SCH28080, pH 4.8 adjusted by Tris buffer. Samples were negatively stained with 2% (w/v) uranyl acetate to screen for crystallization conditions. Sample preparations for cryo-electron microscopy and image processing were as described previously [31] . Briefly, specimens were prepared in the cold room using the carbon sandwich method [36] . Images were recorded with a JEM-3000SFF electron microscope (JEOL) equipped with a super fluid helium stage [32] , [37] on SO-163 film (Kodak). Digitized images were processed with the MRC image processing programme [38] and their initial contrast transfer function parameters were determined [39] for correction. The data tilted to 60° were merged using LATLINE [40] and used to calculate a three-dimensional density map at 7 Å resolution ( Supplementary Table S1 ). Homology modelling and structural analysis The homology model for the H + ,K + -ATPase (SCH)E 2 BeF structure was built with MODELLER v9.7 (ref. 41 ) using the atomic model of ouabain-bound Na + ,K + -ATPase [20] (PDB code 3A3Y ) as a starting template. The initial manual fitting of the homology model into the density map was achieved using the programme O [42] . The adjustment for each individual domain and TM helix with the EM density map was performed using SITUS [43] . After the positional search, further fine fitting and connecting the split loop region were performed manually using O or COOT [44] with regularization refinement. The resulting homology model was consistent with the EM density map ( Fig. 1a ), except in the N-terminal domain and the A-M2 linker of the α-subunit, and in the β-subunit N-terminus and the ectodomain of the β-subunit; these regions were not included in the homology model for the following reasons: (i) The N-terminal domain of the α-subunit was invisible in the EM density map. (ii) The conformation of the A-M2 linker of the EM density map was very different from that in the starting template structure ( Fig. 4 , see also Supplementary Fig. S6 and text ). (iii) The N-terminal tail of the β-subunit was not modelled because of its disorder in the X-ray structures of Na + ,K + -ATPase, in contrast to its strong appearance in the H + ,K + -ATPase EM density map. (iv) The overall structure of the β-subunit ectodomain seemed to be different between the EM density map of the H + ,K + -ATPse and the X-ray structure of the Na + ,K + -ATPase, thus only overlapping parts are shown in the homology model. To determine the SCH28080-binding site clearly, we generated the subtracted density map as follows. Subtraction of the estimated protein density from the EM density map ( Fig. 1b and 2 ) was performed using UCSF Chimera [45] . The volume responsible for the protein part was defined as a 4 Å radius from the backbone chain tracing of the homology model. The whole EM density map, contoured at 1σ, was then subtracted by this assumed protein volume in real space to show the surplus densities. As a result, one significant density is found at the centre of the luminal cavity, corresponding to the bound SCH28080 molecule as described in the results (green mesh in Figs 1b and 2 ). The docking simulation of the SCH28080 was performed using AutoDock Vina [46] . Previous biochemical and mutagenesis studies [22] , [23] , [24] , [25] , [26] , [27] , [28] , [29] suggest that the SCH28080-binding site is located in the cavity facing the gastric lumen. Therefore, the binding search was performed only for the luminal vestibule region (boxed region of 26 Å ( x ) × 20 Å ( y ) × 24 Å ( z ), with C813 centreing). The AUTODOCK Vina programme predicted several binding modes. All of the predicted binding sites were in the luminal cavity, surrounded by A335, Y799 and C813, but with different conformations of SCH28080 binding. Among them, the proposed binding mode had the highest score in this programme and the best fit to the EM density map. See also the Discussion for details. Figures were prepared using UCSF Chimera or Pymol ( http://pymol.sourceforge.net/ ). The EM density map has been deposited in the Macromolecular Structure Database (MSD, http://www.ebi.ac.uk/msd-srv/emsearch/index.html , accession no 1831). The coordinates of the homology model have been deposited in the Protein Data Bank (accession code 2xzb ). How to cite this article: Abe, K. et al . Conformational rearrangement of gastric H + ,K + -ATPase induced by an acid suppressant. Nat. Commun. 2:155 doi: 10.1038/ncomms1154 (2011).